Pin1-dependent signalling negatively affects GABAergic transmission by modulating neuroligin2/gephyrin interaction The cell adhesion molecule Neuroligin2 (NL2) is localized selectively at GABAergic synapses, where it interacts with the scaffolding protein gephyrin in the post-synaptic density. However, the role of this interaction for formation and plasticity of GABAergic synapses is unclear. Here, we demonstrate that endogenous NL2 undergoes proline-directed phosphorylation at its unique S714-P consensus site, leading to the recruitment of the peptidyl-prolyl cis–trans isomerase Pin1. This signalling cascade negatively regulates NL2’s ability to interact with gephyrin at GABAergic post-synaptic sites. As a consequence, enhanced accumulation of NL2, gephyrin and GABA A receptors was detected at GABAergic synapses in the hippocampus of Pin1-knockout mice (Pin1−/−) associated with an increase in amplitude of spontaneous GABA A -mediated post-synaptic currents. Our results suggest that Pin1-dependent signalling represents a mechanism to modulate GABAergic transmission by regulating NL2/gephyrin interaction. Structural and functional changes of post-synaptic density (PSD) components contribute to regulate synapse formation and plasticity. These remodelling events can affect trafficking, lateral mobility and turnover of several classes of structural and signalling molecules. They often involve interactions among specific proteins regulated by post-translational modifications, such as phosphorylation. At GABAergic synapses, the impact of phosphorylation on the gating properties, surface mobility and trafficking of the gamma-aminobutyric acid A receptors (GABA A Rs) has been extensively studied [1] , [2] . Much less is known about the effects of phosphorylation of other post-synaptic proteins functionally linked to GABA A Rs. An important class of molecules involved in synapse formation, maturation and stabilization comprizes the cell adhesion molecules of the neuroligin (NLs) family [3] . These post-synaptic proteins functionally coordinate pre and post-synaptic rearrangements by binding, via their extracellular domain, the presynaptically localized neurexins (NRXs) and via specific intracellular motifs, synapse-specific scaffolding molecules [4] , [5] , [6] . Neuroligin2 (NL2) isoform is the only known adhesion molecule constitutively present at GABAergic PSDs [7] , where it drives the recruitment of inhibitory neurotransmitter receptors as well as the scaffolding molecule gephyrin [6] . Gephyrin, initially identified as a constituent of purified glycine receptor preparations (GlyR) [8] , [9] , was soon recognized a key player in α2 and γ2 subunit-containing GABA A Rs clustering [10] , [11] and to be a central component of the GABAergic (and glycinergic) PSD [8] , [12] . On the basis of its auto-oligomerization properties, gephyrin builds a bidimensional lattice underneath the synaptic membrane, which exposes a high number of binding sites to accumulate GlyR and GABA A Rs in front of the presynaptic releasing sites [13] , [14] , [15] , [16] , [17] . NL2 interacts with gephyrin through a conserved stretch of amino acid residues highly conserved among all family members [6] . Site-directed mutagenesis within this binding module identified a specific tyrosine residue (Y770A) whose alanine substitution impairs NL2 ability to recruit recombinant and endogenous gephyrin to post-synaptic sites [6] . Notably, the corresponding tyrosine residue on NL1, the isoform enriched at excitatory synapses, was found to be phosphorylated in vivo , preventing NL1–gephyrin interaction while favouring PSD95 recruitment at excitatory synapses [18] . Altogether, these findings point to the existence of intracellular signalling mechanisms able to modulate NL-scaffolding protein interactions by modifying specifically NL properties, leading to alteration in excitatory and inhibitory synaptic transmission. In the present study, we have investigated whether post-phosphorylation prolyl-isomerization may affect GABAergic transmission in a similar manner. This signalling cascade targets serine and threonine residues preceding a proline residue to promote conformational changes on its substrate [19] . This effect is achieved by a unique enzyme, peptidyl-prolyl isomerase Pin1, whose catalytic activity facilitates the cis–trans isomerization of the peptide bond [20] , [21] . Notably, Pin1 was found to interact with gephyrin and to alter its overall conformation, thus enhancing its ability to bind the GlyR [22] . Here, we provide evidence that endogenous NL2 can be phosphorylated at its unique Pin1 consensus motif thus rendering it able to physically recruit the phospho-specific effector Pin1. We show that post-phosphorylation prolyl-isomerization can regulate NL2’s ability to complex with gephyrin. Specifically, Pin1-mediated propyl-isomerization of phosphorylated serine 714 negatively modulates NL2–gephyrin complex formation, down-regulating GABAergic synaptic transmission. Endogenous NL2 undergoes proline-directed phosphorylation The cytoplasmic domain (CD) of NL2 possesses a unique consensus motif for proline-directed phosphorylation, S714-P, located 15 amino acids apart from the transmembrane domain ( Fig. 1a ). To assess whether this site can undergo phosphorylation in vivo we used the mitotic phosphoprotein monoclonal 2 (MPM2) antibody that specifically recognizes phosphorylated S/T-P motifs (Davis et al . [23] ). Endogenous NL2 was therefore immunoprecipitated from mouse brain homogenates using an affinity-purified polyclonal antibody raised against its CD or normal mouse IgG as negative control. Western blotting using the MPM2 antibody revealed a band at around 120 kDa that corresponds to the upper band of the doublet recognized by the NL2 antibody in parallel immunoprecipitation experiments ( Fig. 1b ), suggesting that at least a fraction of NL2 can be phosphorylated at its unique Pin1 consensus motif. To demonstrate that phosphorylation at serine 714 is the event responsible for NL2 detection by the MPM2 antibody, we generated the phospho-defective point mutant NL2HA-S714A. This mutation was introduced into a NL2HA hampered in gephyrin binding (NL2HA-S714A-Δgephyrin-binding domain, GBD) (see Supplementary Fig. 1 ), to exclude the possibility that the MPM2 antibody would immune-react with phosphorylated Pin1 consensus motifs on endogenous gephyrin, which is, at the same time, a Pin1 target [22] and an interacting partner of NL2 (ref. 6 ). Under these conditions, the MPM2 antibody efficiently immunoprecipitated only NL2HA-ΔGBD but not the corresponding point mutant, as indicated by the anti-HA immunoblot ( Fig. 1c ), thus demonstrating that S714 can be found phosphorylated on NL2. 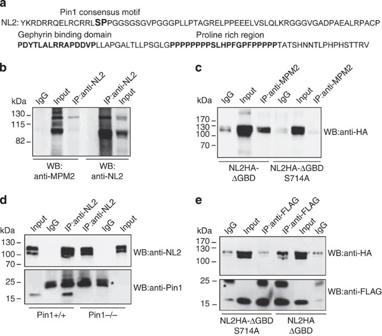Figure 1: NL2 is a proline-directed substrate. (a) Amino acid sequence of the NL2 CD. In bold is marked the unique Pin1 consensus motif (S714-P). The gephyrin-binding domain and the proline-rich region are highlighted in bold. (b) Representative immunoblotting of endogenous NL2 immunoprecipitated (IP) from mouse brain and probed with the anti-MPM2 that specifically recognizes phosphorylated S/T-P motifs and anti-NL2. Rabbit IgGs were used as negative control (IgG) (n=4). (c) Representative immunoblotting of overexpressed NL2HA lacking the gephyrin binding domain (NL2HA-ΔGBD) and the corresponding point mutant (NL2HA-ΔGBDSer714Ala) immunoprecipitated by the phospho-specific MPM2 antibody. Western blot analysis was carried out with anti-HA monoclonal antibody. Mouse IgGs were used as negative control (n=5). (d) Co-immunoprecipitation (Co-IP) of endogenous NL2 and Pin1 from DSP cross-linked brain homogenates of Pin1+/+ or Pin1−/− mice. Western blots were performed with anti-NL2 polyclonal and anti-Pin1 monoclonal antibodies. Mouse IgGs were used as negative control. Asterisk indicate the IgG light chains (n=6). (e) FLAG epitopes from cross-linked samples of HEK293 cells co-expressing Pin1-FLAG and NL2HA-ΔGBD or NL2HA-ΔGBDS714 were immunoprecipitated by anti-FLAG antibody. Western blot was performed with anti-HA and anti-FLAG monoclonal antibodies. Mouse IgGs were used as negative control (n=4). Full images of western blots are inSupplementary Fig. 5. Figure 1: NL2 is a proline-directed substrate. ( a ) Amino acid sequence of the NL2 CD. In bold is marked the unique Pin1 consensus motif (S714-P). The gephyrin-binding domain and the proline-rich region are highlighted in bold. ( b ) Representative immunoblotting of endogenous NL2 immunoprecipitated (IP) from mouse brain and probed with the anti-MPM2 that specifically recognizes phosphorylated S/T-P motifs and anti-NL2. Rabbit IgGs were used as negative control (IgG) ( n =4). ( c ) Representative immunoblotting of overexpressed NL2HA lacking the gephyrin binding domain (NL2HA-ΔGBD) and the corresponding point mutant (NL2HA-ΔGBDSer714Ala) immunoprecipitated by the phospho-specific MPM2 antibody. Western blot analysis was carried out with anti-HA monoclonal antibody. Mouse IgGs were used as negative control ( n =5). ( d ) Co-immunoprecipitation (Co-IP) of endogenous NL2 and Pin1 from DSP cross-linked brain homogenates of Pin1+/+ or Pin1−/− mice. Western blots were performed with anti-NL2 polyclonal and anti-Pin1 monoclonal antibodies. Mouse IgGs were used as negative control. Asterisk indicate the IgG light chains ( n =6). ( e ) FLAG epitopes from cross-linked samples of HEK293 cells co-expressing Pin1-FLAG and NL2HA-ΔGBD or NL2HA-ΔGBDS714 were immunoprecipitated by anti-FLAG antibody. Western blot was performed with anti-HA and anti-FLAG monoclonal antibodies. Mouse IgGs were used as negative control ( n =4). Full images of western blots are in Supplementary Fig. 5 . Full size image The essential feature of proline-directed phosphorylation as a signalling mechanism relies on the ability of phosphorylated S/T-P motifs to recruit the prolyl isomerase Pin1 (refs 19 , 24 ). To test whether this unique phospho-epitope is able to recruit the effector molecule of the signalling cascade, we performed co-immunoprecipitation experiments from Pin1+/+ and Pin1−/− brain lysates. This approach unveiled that Pin1 can be detected in NL2, but not in control, immunoprecipitates or in the absence of Pin1 expression ( Fig. 1d ). To exclude the possibility that Pin1 co-precipitated by NL2 is bound to endogenous gephyrin, these assays were performed on co-expression of NL2HA-ΔGBD and Pin1-FLAG in HEK293 cells. Cell lysates were immunoprecipitated with the anti-FLAG antibody and bound protein complexes analysed by western blotting using anti-HA and anti-FLAG antibodies for NL2 and Pin1 detection, respectively. As shown in Fig. 1e , while NL2HA-ΔGBD was still able to be immunoprecipitated from cells expressing Pin1-FLAG, S714 to alanine mutagenesis completely abolished such interaction, indicating that S714 represents a newly identified Pin1 target. Pin1 modulates gephyrin–NL2 interaction The observation that two fundamental components of the GABAergic PSD are both targets of proline-directed phosphorylation prompted us to investigate whether such signalling cascade would modulate their interaction. To this end, we initially co-expressed gephyrin-FLAG and NL2HA in HEK293 cells and examined the amount of NL2HA that complex with gephyrin-FLAG at 48 h after treating the cells with the selective and reversible inhibitor of Pin1 isomerase activity PiB (IC 50 of approximately 1.5 μM) (ref. 25 ). As shown in Fig. 2a , even though the anti-FLAG antibody immunoprecipitated comparable amounts of gephyrin-FLAG, a significant increase (64%) in the amount of co-precipitated NL2HA was observed on PiB treatment as compared with mock-treated cells (dimethylsulfoxide, DMSO). Interestingly, a marked increase (140%) was detected on gephyrin-FLAG co-precipitation by NL2HA-S714A as compared with NL2HA, indicating that Pin1 exerts a negative control on NL2–gephyrin complex formation, at least in part, through NL2 prolyl-isomerization ( Fig. 2b ). 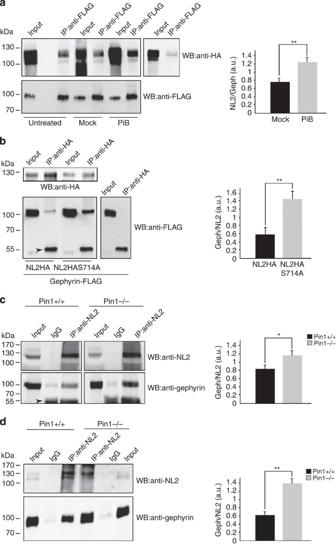Figure 2: Pin1 negatively modulates NL2/gephyrin interaction. (a) Representative IP of FLAG epitopes from samples of HEK293 cells co-expressing gephyrin-FLAG and NL2HA and treated for 48 h with PiB 2.5 μM, DMSO (mock) or untreated. IP was also performed on NL2HA single transfected cells as a negative control. Nitrocellulose membranes were probed with anti-HA and anti-FLAG antibodies. The histogram on the right shows the relative amount of NL2 co-precipitated by gephyrin-FLAG in control and PiB treated cells obtained from densitometric analysis (n=5, mean values±s.d., **P<0.001, Student’st-test). (b) Lysates of HEK cells transfected with gephyrin-FLAG in the presence of NL2HA or NL2HA-S714A or with gephyrin alone (as a negative control) were immunoprecipitated with anti-HA agarose. Immunoprecipitates were analysed by western blotting using anti-FLAG and anti-HA monoclonal antibodies. Arrowhead indicates the IgG heavy chains. The histogram on the right shows the relative amount of gephyrin-FLAG in complex with either NL2HA or NL2HA-S714A co-precipitated by anti-HA agarose obtained from densitometric analysis (n=5, mean values±s.d., **P<0.001, Student’st-test). (c) Co-IP of endogenous NL2/gephyrin complexes from DSP cross-linked brain homogenates of Pin1+/+ or Pin1−/− mice. Western blots were performed with anti-NL2 polyclonal and anti-gephyrin monoclonal antibodies. Rabbit IgGs were used as negative control. An increased amount of gephyrin co-precipitates in complex with NL2 in the absence of Pin1 expression. Arrowhead indicates the IgG heavy chains. The histogram on the right shows the relative amount (obtained from densitometric analysis) of endogenous gephyrin co-precipitated by endogenous NL2 from both mouse genotypes (n=8, mean values±s.d., *P<0.01, Student’st-test). (d) A similar experiment described incwas carries out on hippocampus isolated from of Pin1+/+ or Pin1−/− mice. The histogram on the right shows the relative amount (obtained from densitometric analysis) of endogenous gephyrin co-precipitated by endogenous NL2 from both mouse genotypes (n=4, mean values±s.d., **P<0.001, Student’st-test). Full images of western blots are inSupplementary Fig. 5. Figure 2: Pin1 negatively modulates NL2/gephyrin interaction. ( a ) Representative IP of FLAG epitopes from samples of HEK293 cells co-expressing gephyrin-FLAG and NL2HA and treated for 48 h with PiB 2.5 μM, DMSO (mock) or untreated. IP was also performed on NL2HA single transfected cells as a negative control. Nitrocellulose membranes were probed with anti-HA and anti-FLAG antibodies. The histogram on the right shows the relative amount of NL2 co-precipitated by gephyrin-FLAG in control and PiB treated cells obtained from densitometric analysis ( n =5, mean values±s.d., ** P <0.001, Student’s t -test). ( b ) Lysates of HEK cells transfected with gephyrin-FLAG in the presence of NL2HA or NL2HA-S714A or with gephyrin alone (as a negative control) were immunoprecipitated with anti-HA agarose. Immunoprecipitates were analysed by western blotting using anti-FLAG and anti-HA monoclonal antibodies. Arrowhead indicates the IgG heavy chains. The histogram on the right shows the relative amount of gephyrin-FLAG in complex with either NL2HA or NL2HA-S714A co-precipitated by anti-HA agarose obtained from densitometric analysis ( n =5, mean values±s.d., ** P <0.001, Student’s t -test). ( c ) Co-IP of endogenous NL2/gephyrin complexes from DSP cross-linked brain homogenates of Pin1+/+ or Pin1−/− mice. Western blots were performed with anti-NL2 polyclonal and anti-gephyrin monoclonal antibodies. Rabbit IgGs were used as negative control. An increased amount of gephyrin co-precipitates in complex with NL2 in the absence of Pin1 expression. Arrowhead indicates the IgG heavy chains. The histogram on the right shows the relative amount (obtained from densitometric analysis) of endogenous gephyrin co-precipitated by endogenous NL2 from both mouse genotypes ( n =8, mean values±s.d., * P <0.01, Student’s t -test). ( d ) A similar experiment described in c was carries out on hippocampus isolated from of Pin1+/+ or Pin1−/− mice. The histogram on the right shows the relative amount (obtained from densitometric analysis) of endogenous gephyrin co-precipitated by endogenous NL2 from both mouse genotypes ( n =4, mean values±s.d., ** P <0.001, Student’s t -test). Full images of western blots are in Supplementary Fig. 5 . Full size image This issue was then investigated using a source of native NL2–gephyrin complexes mouse brain homogenates from both genotypes. For these experiments, endogenous NL2 was immunoprecipitated using a rabbit polyclonal anti-NL2 antibody and the co-precipitated gephyrin fraction was visualized by the monoclonal 3B11 antibody ( Fig. 2c ). In the absence of Pin1 expression, the amount of gephyrin co-precipitated by NL2 was increased by 40% as compared with Pin1 expressing neurons. This approach was also applied on hippocampal tissues isolated from both mouse genotypes. Here, the enrichment of gephyrin co-precipitated by NL2 in the absence of Pin1 expression was even more dramatic as compared with the amount detected from whole brain (130% increase; Fig. 2d ), suggesting a strong impact of such signalling pathway on GABAergic synapses of the hippocampus. Characterization of gephyrin Pin1 sites S270-P and S319-P The scaffolding molecule gephyrin possesses 10 putative Pin1 consensus motifs, the majority of them being concentrated in the central region (C-domain) [26] . To determine whether specific Pin1 sites may contribute to enhance NL2/gephyrin complex formation, we decided to focus on those located close to, or within, the NL2 binding site on gephyrin. A previous yeast two-hybrid screening identified a large portion of gephyrin encompassing the E-domain and part of the C-domain as the region involved in NL2 interaction [6] . We re-examine this issue by generating eGFP-tagged gephyrin truncated version to be tested in GST-NL2-CD pulldown assays. HEK293 cells transfected with different eGFP-gephyrin variants were incubated with GST-NL2-CD loaded beads or with GST alone as negative controls. As shown in Fig. 3a , while gephyrin 310–736 was recruited even better than the wild-type (WT) version, the mutants gephyrin 326–736 and gephyrin 1–310 (gephyrin GC) displayed a reduced binding activity as compared to both gephyrin full-length (FL) and the truncated version 310–736 ( Fig. 3a ). Since the two E-domain gephyrin versions, showing such a striking difference in the binding affinity, differ only for a short stretch of amino acids, we generated the deletion mutant removing, from the FL protein, only the residues contained in this region but belonging to the E-domain itself (gephyrinΔ319–329) and assayed it for NL2 binding. Interestingly, the lack of this short sequence almost completely abolished the interaction of gephyrin with NL2 ( Fig. 3b ), indicating that epitope(s) contained in the C-domain together with this minimal binding module are involved in gephyrin recruitment. 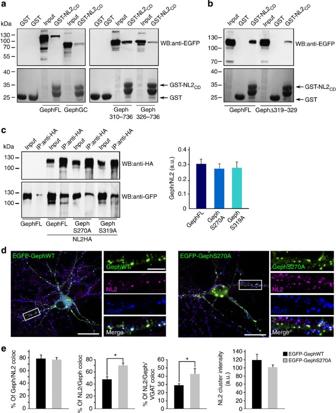Figure 3: Impact of gephyrin S270A and S319A in NL2/gephyrin interaction. (a) GST-NL2-CD pulldown from samples of HEK293 expressing EGFP-gephyrin full-length (FL), EGFP-gephyrin 310–736 (E-310), EGFP-gephyrin 326–736 (E-326) and EGFP-gephyrin GC. GST was used as negative control. Pulled down eGFPgephyrin variants were detected using an anti-GFP monoclonal antibody. The bottom panels show the levels of GST and GST-NL2-CD in the pulldown assays (Ponceau staining) (n=8). (b) EGFP-gephyrin Δ319 to 329 was tested in similar pulldown assays. Western blots inaandbwere performed using anti-GFP antibody. Gephyrin requires amino acid sequence 319–329 for its efficient recruitment by NL2 (n=6). (c) Representative IP of HA epitopes from samples of HEK293 cells co-expressing NL2HA and EGFP-gephyrin WT, EGFP-gephyrinS270A or EGFP-gephyrinS319A. Nitrocellulose membranes were probed with anti-HA and anti-GFP antibodies. EGFP-gephyrin single transfected cells incubated with HA agarose were used as negative controls. The histogram on the right shows the relative amount of eGFP-gephyrinWT and point mutants co-precipitated by NL2HA (n=4, mean values±s.d.,P>0.05). (d) Representative images of hippocampal neurons transfected with EGFP-gephyrin and EGFP-gephyrinS270A point mutant immunolabeled for endogenous NL2 (magenta) and VGAT (blue) at DIV10. Enlarged boxed areas are shown aside to the corresponding full view image. Post-synaptic clustering is demonstrated by apposition of gephyrin/NL2 clusters to VGAT positive terminals on the merge window. Scale bars, 20 μm in full view images and 5 μm in enlarged panels. (e) Distribution histograms of the % of gephyrin clusters colabeled with NL2 (79±5% in EGFP-gephyrinWT versus 77±4% in EGFP-gephyrinS270A), % of NL2 clusters colabeled with gephyrin (48±5% in EGFP-gephyrinWT versus 71±4% in EGFP-gephyrinS270A), % of NL2 synaptically localized (29±2% in EGFP-gephyrinWT versus 43±6% in EGFP-gephyrinS270A) and NL2 clusters intensity (119±15 a.u. in EGFP-gephyrinWT versus 102 a.u.±6 in EGFP-gephyrinS270A). The number of transfected hippocampal neurons investigated in each experiments (four independent experiments) were as follow:n=15 for eGFP-gephyrinWT,n=10 for eGFP-gepyrinS270A (for each neurons at least 4 dendritic regions of interests were measured, mean values±s.d., *P<0.01, Student’st-test). Figure 3: Impact of gephyrin S270A and S319A in NL2/gephyrin interaction. ( a ) GST-NL2-CD pulldown from samples of HEK293 expressing EGFP-gephyrin full-length (FL), EGFP-gephyrin 310–736 (E-310), EGFP-gephyrin 326–736 (E-326) and EGFP-gephyrin GC. GST was used as negative control. Pulled down eGFPgephyrin variants were detected using an anti-GFP monoclonal antibody. The bottom panels show the levels of GST and GST-NL2-CD in the pulldown assays (Ponceau staining) ( n =8). ( b ) EGFP-gephyrin Δ319 to 329 was tested in similar pulldown assays. Western blots in a and b were performed using anti-GFP antibody. Gephyrin requires amino acid sequence 319–329 for its efficient recruitment by NL2 ( n =6). ( c ) Representative IP of HA epitopes from samples of HEK293 cells co-expressing NL2HA and EGFP-gephyrin WT, EGFP-gephyrinS270A or EGFP-gephyrinS319A. Nitrocellulose membranes were probed with anti-HA and anti-GFP antibodies. EGFP-gephyrin single transfected cells incubated with HA agarose were used as negative controls. The histogram on the right shows the relative amount of eGFP-gephyrinWT and point mutants co-precipitated by NL2HA ( n =4, mean values±s.d., P> 0.05). ( d ) Representative images of hippocampal neurons transfected with EGFP-gephyrin and EGFP-gephyrinS270A point mutant immunolabeled for endogenous NL2 (magenta) and VGAT (blue) at DIV10. Enlarged boxed areas are shown aside to the corresponding full view image. Post-synaptic clustering is demonstrated by apposition of gephyrin/NL2 clusters to VGAT positive terminals on the merge window. Scale bars, 20 μm in full view images and 5 μm in enlarged panels. ( e ) Distribution histograms of the % of gephyrin clusters colabeled with NL2 (79±5% in EGFP-gephyrinWT versus 77±4% in EGFP-gephyrinS270A), % of NL2 clusters colabeled with gephyrin (48±5% in EGFP-gephyrinWT versus 71±4% in EGFP-gephyrinS270A), % of NL2 synaptically localized (29±2% in EGFP-gephyrinWT versus 43±6% in EGFP-gephyrinS270A) and NL2 clusters intensity (119±15 a.u. in EGFP-gephyrinWT versus 102 a.u.±6 in EGFP-gephyrinS270A). The number of transfected hippocampal neurons investigated in each experiments (four independent experiments) were as follow: n =15 for eGFP-gephyrinWT, n =10 for eGFP-gepyrinS270A (for each neurons at least 4 dendritic regions of interests were measured, mean values±s.d., * P <0.01, Student’s t -test). Full size image On the basis of these results, two Pin1 consensus sites were further characterized, namely S319-P, located at the edge of the minimal binding module, and S270-P, positioned in its proximity, still contained, in the C-domain participating in NL2 binding. To this end, we introduced point mutations in eGFP-gephyrin to create S319A and S270A mutants and tested them for their ability to interact with NL2HA. As judged by co-immunoprecipitation experiments, no significant differences were observed in binding capacity of the mutants as compared with gephyrin WT ( Fig. 3c ). These constructs were also overexpressed in cultured hippocampal neurons to analyse and quantify their impact on endogenous NL2 distribution using immunofluorescence staining and confocal microscopy. As previously reported, neurons expressing the S270A mutants had an increased number, unchanged in size, of gephyrin clusters compared with eGFP-gephyrin WT [27] (18.9±1.7 per 20 μm dendritic segment versus 6.5±0.6, P =0.00015). The expression of the S319A construct produced a dramatic decrease in cluster density associated with a diffuse cytoplasmic staining. This latter effect seems to correlate with the intrinsic instability of the mutant protein that undergoes a high rate of degradation on neuronal expression (data not shown), hampering its further characterization. Clusters formed by gephyrin S270A co-localized with NL2 at the same extent as the WT protein (around 78%; Fig. 3d,e ). The fraction of NL2 clusters co-localizing with S270A mutant as well as their synaptic localization were increased as compared with gephyrin WT but their intensity values (calculated by normalizing cluster fluorescence intensity to cluster area and expressed in a.u. : 119 a.u.±15.2 versus 102±6.3) were unchanged ( Fig. 3e ). These data indicate that the increase in NL2/gephyrin S270 interaction observed by immunoprecipitation is simply due to the augmented S270A cluster density and not to an enhance affinity of the mutant for NL2. Pin1 selectively controls NL2 synaptic enrichment Pin1 has emerged as a negative regulator of gephyrin–NL2 interaction. Since these protein complexes are mainly localized at the plasma membrane, we tested whether Pin1 affects the amount of NL2 transported to, or maintained at, the neuronal plasma membrane. To this end, cultured hippocampal neurons derived from Pin1+/+ and Pin1−/− mice were subjected to surface biotinylation assay. Cell surface proteins were treated with the membrane-impermeant sulfo-NHS-biotin reagent, then isolated by binding to Streptavidin beads and probed with anti-NL2 antibody. To check for unspecific protein binding during surface biotinylation experiments, hippocampal neurons not labelled with biotin were processed with biotinylated samples. Western blot detecting the intracellular glycophosphatidylinositol-anchored protein Flotilin1 was included to ensure that similar amount of associated membrane proteins, biotinylated or not, where incubated with Streptavidin beads. No major differences on the total content of membrane localized NL2 were observed between Pin1+/+ and Pin1−/− ( Fig. 4a ). 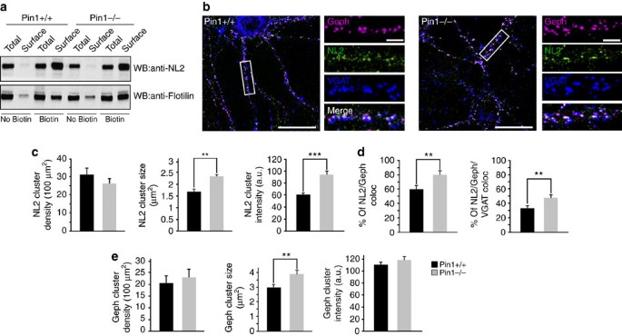Figure 4: Pin1 enhances NL2 synaptic content not its surface abundance. (a) Surface NL2 derived from cultured hippocampal neurons of Pin1+/+ and Pin1−/− mice was isolated by biotinylation assay and detected by anti-NL2 antibody. No biotinylated neuronal cells were processed in parallel to evaluate unspecific NL2 binding. Western blot detecting glycophosphatidylinositol-anchored Flotilin was used as loading control (n=4). Full images of western blots are inSupplementary Fig. 5. (b) Typical examples of hippocampal neurons from Pin1+/+ and Pin1−/− immunolabeled for endogenous gephyrin (magenta), NL2 (green) and VGAT (blue) at DIV10. Enlarged boxed areas are shown aside to the corresponding full view image. Post-synaptic clustering is demonstrated by apposition of gephyrin/NL2 clusters to VGAT positive terminals on the merge window. Scale bars, 20 μm in full view images and 5 μm in enlarged panels. (c) Distribution histograms of NL2 cluster density (normalized to 100 μm2), the average cluster size and intensity in Pin1+/+ and Pin1−/− hippocampal neurons. (d) Distribution histograms of the percentage of NL2 co-localizing with gephryin and the percentage of double labelled NL2/gephyrin puncta overlapping with the presynaptic marker VGAT. (e) Distribution histograms of gephyrin cluster density (normalized to 100 μm2), the average cluster size and intensity (calculated as described inc) in both mouse genotypes. The number of hippocampal neurons investigated in each experiments (three independent experiments) were as follows:n=10 for Pin1+/+,n=12 for Pin1−/−. For each neurons, at least five dendritic regions of interests were measured, mean values±s.d., **P<0.001, ***P<0.0001, Student’st-test). Figure 4: Pin1 enhances NL2 synaptic content not its surface abundance. ( a ) Surface NL2 derived from cultured hippocampal neurons of Pin1+/+ and Pin1−/− mice was isolated by biotinylation assay and detected by anti-NL2 antibody. No biotinylated neuronal cells were processed in parallel to evaluate unspecific NL2 binding. Western blot detecting glycophosphatidylinositol-anchored Flotilin was used as loading control ( n =4). Full images of western blots are in Supplementary Fig. 5 . ( b ) Typical examples of hippocampal neurons from Pin1+/+ and Pin1−/− immunolabeled for endogenous gephyrin (magenta), NL2 (green) and VGAT (blue) at DIV10. Enlarged boxed areas are shown aside to the corresponding full view image. Post-synaptic clustering is demonstrated by apposition of gephyrin/NL2 clusters to VGAT positive terminals on the merge window. Scale bars, 20 μm in full view images and 5 μm in enlarged panels. ( c ) Distribution histograms of NL2 cluster density (normalized to 100 μm 2 ), the average cluster size and intensity in Pin1+/+ and Pin1−/− hippocampal neurons. ( d ) Distribution histograms of the percentage of NL2 co-localizing with gephryin and the percentage of double labelled NL2/gephyrin puncta overlapping with the presynaptic marker VGAT. ( e ) Distribution histograms of gephyrin cluster density (normalized to 100 μm 2 ), the average cluster size and intensity (calculated as described in c ) in both mouse genotypes. The number of hippocampal neurons investigated in each experiments (three independent experiments) were as follows: n =10 for Pin1+/+, n =12 for Pin1−/−. For each neurons, at least five dendritic regions of interests were measured, mean values±s.d., ** P <0.001, *** P <0.0001, Student’s t -test). Full size image These results allow excluding the involvement of Pin1 in NL2 transport and/or turnover at the plasma membrane. Surface biotinylation represents an experimental approach that cannot provide an accurate analysis of protein distributions among different membrane domains. Since NL2 is enriched at GABAergic synapses, but is also distributed on extrasynaptic sites [28] , with this approach differences in NL2 partitioning between these two compartments might have been missed. To this aim, immunocytochemical experiments were performed in dissociated Pin1+/+ and Pin1−/− hippocampal neurons co-labelled for NL2, gephyrin and VGAT, a specific marker of GABAergic innervations [29] ( Fig. 4b ). In the absence of Pin1 expression a significant increase in NL2 cluster size (2.4 μm 2 ±0.2 versus 1.7 μm 2 ±0.2, P =0.00044) and intensity (92 a.u.±4.0 versus 58 a.u.±2, P <0.00048) was observed as compared with WT neurons, while no major changes in NL2 cluster density were detected ( Fig. 4c ). The fraction of NL2-positive clusters co-localized with endogenous gephyrin puncta was also enhanced in Pin1−/− cells (80±3.0% versus 60±5%, P =0.00013) and found enriched at post-synaptic sites, as demonstrated by the higher percentage of NL2/gephyrin co-stained puncta overlapping with the presynaptic marker VGAT (48±4% versus 33±4%, P =0.0008; Fig. 4d ). Gephyrin puncta appeared slightly, but significantly, increased in size while their density and intensity values were unchanged as compared with Pin1+/+ ( Fig. 4e ). These observations suggest that the absence of Pin1 promotes the formation and/or stabilization of NL2/gephyrin complexes at GABAergic post-synaptic sites. NL2/gephyrin complex modulates synaptic abundance of GABA A Rs The recruitment of GABA A Rs at synaptic sites is functionally coupled to NLs expression levels as well as to the gephyrin scaffold [6] . To assess whether the enhanced NL2/gephyrin complex formation detected at GABAergic synapses similarly affects the distribution of synaptic γ2 subunit-containing GABA A Rs, we performed a quantitative evaluation of the γ2 subunit present in synaptosome suspensions isolated from the hippocampus of Pin1+/+ and Pin1−/− mice. Quantitative immunoblot analysis was also extended to NL2 and gephyrin to further verify their synaptic enrichment. As shown in Fig. 5a , the amount of all three markers investigated was significant increased in Pin1−/− mice as compared with Pin1+/+. The synaptic enrichment (synaptic fraction versus homogenate) was 35±5% for the NL2, 30±6% for the γ2 subunit and 20±4% for gephyrin. 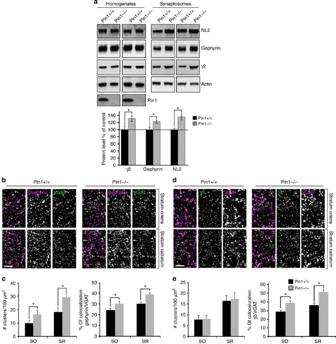Figure 5: Synaptic enrichment of GABAARs is achieved in Pin1−/−. (a) Representative immunoblots of NL2, gephyrin and γ2 subunit of GABAAreceptor extracted from the hippocampus of Pin1+/+ and Pin1−/− mice (littermates) in two different sets of experiments. Total proteins from the homogenates and synaptosome suspension fractions were analysed by western blotting. Below: quantification of the indicated antigens extracted from hippocampal tissues of Pin1+/+ and Pin1−/− mice. All markers analysed are enriched at inhibitory synapses. Western blot to actin was done as loading control. Pin1 immunoblot indicates hyppocampus from Pin1+/+ and Pin1−/− (n=6 littermate pairs, mean values±s.d, *P<0.05, Student’st-test) Full images of western blots are inSupplementary Fig. 5. (b) Representative confocal micrographs of frontal brain sections showing segments of the SR and SO of the CA1 region of the hippocampus from adult Pin1+/+ and Pin1−/− mice immunolabeled for gephyrin (magenta) and VGAT (green). Scale bar, 5 μm. (c) Quantification of gephyrin punctum density (normalized to 100 μm2) and their percentage of colocalization with the presynaptic marker VGAT in both mouse genotypes. (d) Confocal micrographs as inaimmunolabeled for GABAAreceptor γ2 subunit (green) and VGAT (magenta). (e) Quantification of γ2 subunit punctum and their percentage of colocalization with VGAT in both mouse genotypes. The number of gephyrin, γ2, gephyrin and VGAT puncta was assessed in at least eight sections for each genotypes (Pin1+/+ and Pin1−/−), by taking at least four images of SR and SO of the CA1 region of each hippocampus in each set of experiments (n=3). Mean values±s.d., *P<0.05, Student’st-test. Scale bar, 5 μm. Figure 5: Synaptic enrichment of GABA A Rs is achieved in Pin1−/−. ( a ) Representative immunoblots of NL2, gephyrin and γ2 subunit of GABA A receptor extracted from the hippocampus of Pin1+/+ and Pin1−/− mice (littermates) in two different sets of experiments. Total proteins from the homogenates and synaptosome suspension fractions were analysed by western blotting. Below: quantification of the indicated antigens extracted from hippocampal tissues of Pin1+/+ and Pin1−/− mice. All markers analysed are enriched at inhibitory synapses. Western blot to actin was done as loading control. Pin1 immunoblot indicates hyppocampus from Pin1+/+ and Pin1−/− ( n =6 littermate pairs, mean values±s.d, * P <0.05, Student’s t -test) Full images of western blots are in Supplementary Fig. 5 . ( b ) Representative confocal micrographs of frontal brain sections showing segments of the SR and SO of the CA1 region of the hippocampus from adult Pin1+/+ and Pin1−/− mice immunolabeled for gephyrin (magenta) and VGAT (green). Scale bar, 5 μm. ( c ) Quantification of gephyrin punctum density (normalized to 100 μm 2 ) and their percentage of colocalization with the presynaptic marker VGAT in both mouse genotypes. ( d ) Confocal micrographs as in a immunolabeled for GABA A receptor γ2 subunit (green) and VGAT (magenta). ( e ) Quantification of γ2 subunit punctum and their percentage of colocalization with VGAT in both mouse genotypes. The number of gephyrin, γ2, gephyrin and VGAT puncta was assessed in at least eight sections for each genotypes (Pin1+/+ and Pin1−/−), by taking at least four images of SR and SO of the CA1 region of each hippocampus in each set of experiments ( n =3). Mean values±s.d., * P <0.05, Student’s t -test. Scale bar, 5 μm. Full size image We also examined the number of puncta labelled for gephyrin and γ2 subunit-specific antibodies, as well as their levels of colocalization with the presynaptic marker VGAT, in the CA1 region of the hippocampus of both genotypes. The staining pattern of gephyrin in Pin1−/− demonstrated a slight increase in the number of clusters both in the stratum oriens (SO) and stratum radiatum (SR) as compared with Pin1+/+ (SO 16±3 clusters per 100 μm 2 and SR 28±3 clusters per 100 μm 2 versus SO 10±2 clusters per 100 μm 2 and SR 19±3 clusters per 100 μm 2 ; P <0.05; Fig. 5b,c ). This increase was paralleled by a small increase (around 6–8%) in gephyrin puncta co-localized with presynaptic VGAT (SO 30±2% and SR 39±1.4% versus SO 24±2% and SR 31±2%; P <0.05; Fig. 5b,c ). The average cluster size and intensity were similar in both genotypes (3.6 μm 2 ±0.2 versus 3.5 μm 2 ±0.3 and 61±7 versus 65±4 a.u. for cluster size and intensity in Pin1−/− versus Pin1+/+, respectively). The γ2 subunit staining pattern exhibited a similar cluster density in the two strata analysed in both genotypes (SO 8±2 and SR 18±2 versus SO 8±1 and SR 17±1.2; P> 0.05; Fig. 5d,e ). A small, although significant, increase in their intensity was evident (120±3 RFU versus 106±2 RFU in Pin1−/− versus Pin1+/+; P <0.05) but they were similar in size (4.3 μm 2 ±0.5 versus 3.7 μm 2 ±0.5). VGAT colocalization was increased by 10–15% in tissue from knockout animals (SO 38.9±2.7% and SR 52±3% versus SO 29±2% and SR 36±3%; P <0.05; Fig. 5d,e ). The changes in gephyrin and γ2 subunit synaptic fraction are not due to an increase in synapses numbers, the density of inhibitory terminals being unaltered between the two genotypes, as assessed by quantification of VGAT immunolabeling (SO 14±2% and SR 22±3% versus SO 13±2% and SR 21±3%; P >0.05). Altogether, these data indicate that the enhanced interaction between gephyrin and NL2 observed in the absence of Pin1 is associated with a concomitant increase in the synaptic recruitment of γ2 subunit-containing GABA A Rs. Pin1 signalling affects the number of synaptic GABA A Rs To functionally explore whether the enrichment of γ2 subunit-containing GABA A Rs in Pin1−/− mice affects GABAergic transmission, whole-cell recordings in voltage clamp configuration were performed from CA1 principal cells in hippocampal slices obtained from Pin1+/+ and Pin1−/− mice at postnatal (P) day P10–P13. These neurons presented similar resting membrane potential ( V rest ) and input resistance ( R in ) values (data not shown), thus indicating that Pin1 does not affect the passive membrane properties of principal cells. Spontaneous GABA A -mediated inhibitory post-synaptic currents (sIPSCs) were then recorded from both genotypes in the presence of 6,7-dinitroquinoxaline-2,3-dione (DNQX; 20 μM) to block AMPA-mediated excitatory post-synaptic currents (sEPSCs). As shown in Fig. 6a , recordings from Pin1−/− mice exhibited sIPSCs of higher amplitude values compared with control littermates (106±12 pA versus 62±8 pA; P <0.05), in the absence of any significant change in frequency (4.2±0.5 Hz versus 3.6±0.6 Hz; P >0.05; Fig. 6b ). The amplitude distribution histogram of sIPSCs recorded in Pin1−/− unveiled a clear peak at ~200 pA ( Fig. 6c ). The observed effects were selective for sIPSCs since no significant differences in amplitude (22±2 pAin Pin1−/− mice and 27±4 pA in Pin1+/+; n =6 for both genotypes; P >0.05) or frequency (1.7±0.3 Hz in Pin1−/− mice and 1.3±0.4 Hz in Pin1+/+ mice; P >0.05) of sEPSCs (recorded in the presence of picrotoxin, PTX, 100 μM) were detected between the two genotypes ( Supplementary Fig. 2a,b ). 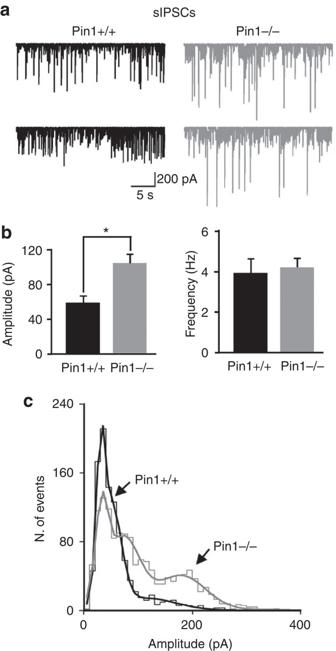Figure 6: Pin1 affects the amplitude but not the frequency of sIPSCs. (a) Representative traces of sIPSCs recorded from CA1 principal cells at P11 in hippocampal slices from Pin1+/+ (black) and Pin1−/− mice (grey). Note higher amplitude events in Pin1−/− mice. (b) Each column represents the mean frequency and amplitude values of sIPSCs recorded from Pin1+/+ (black,n=9) and Pin−/− mice (grey,n=8). *P<0.05, Student’st-test). (c) Amplitude distribution histograms of sIPSCs recorded in Pin1+/+ (1,030 events; black) and in Pin1−/− mice (1,412 events; grey). Note the appearance of a clear peak at ~200 pA in Pin1−/− mice. Figure 6: Pin1 affects the amplitude but not the frequency of sIPSCs. ( a ) Representative traces of sIPSCs recorded from CA1 principal cells at P11 in hippocampal slices from Pin1+/+ (black) and Pin1−/− mice (grey). Note higher amplitude events in Pin1−/− mice. ( b ) Each column represents the mean frequency and amplitude values of sIPSCs recorded from Pin1+/+ (black, n =9) and Pin−/− mice (grey, n =8). * P <0.05, Student’s t -test). ( c ) Amplitude distribution histograms of sIPSCs recorded in Pin1+/+ (1,030 events; black) and in Pin1−/− mice (1,412 events; grey). Note the appearance of a clear peak at ~200 pA in Pin1−/− mice. Full size image Spontaneous inhibitory events from hippocampal neurons in culture overexpressing the NL2HA-S714A mutation exhibited, compared with NL2HA-transfected cells, a significant increase in amplitude (but not frequency), which in part mimicked the phenotype observe in Pin1−/− mice, suggesting that the interaction of Pin1 with NL2 is critical for this effect ( Fig. 7a ). As shown in the cumulative amplitude plot ( Fig. 7b ), the curve obtained from NL2HA-S714A transfected cells was shifted to the right as compared with cells expressing NL2HA ( P <0.05). 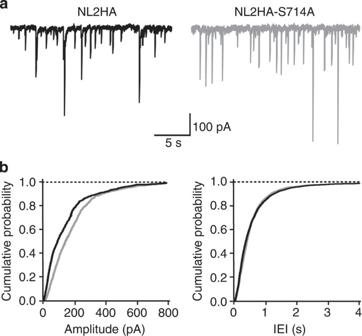Figure 7: Changes in amplitude of sIPSCs involve the interaction of Pin1 with NL2. (a) Samples traces of sIPSCs recorded from hippocampal neurons in culture expressing either the NL2HA or the NL2HA-S714A mutation. (b) Amplitude and inter-event interval (IEI) plots of sIPSCs recorded in cells transfected either with the NL2HA (black;n=7) or the NL2HA-S714A point mutant (grey;n=12).P<0.05; Kolmogorov–Smirnov test. Note the shift to the right of the cumulative amplitude distribution curve obtained from cells transfected with the mutant as compared to controls. Figure 7: Changes in amplitude of sIPSCs involve the interaction of Pin1 with NL2. ( a ) Samples traces of sIPSCs recorded from hippocampal neurons in culture expressing either the NL2HA or the NL2HA-S714A mutation. ( b ) Amplitude and inter-event interval (IEI) plots of sIPSCs recorded in cells transfected either with the NL2HA (black; n =7) or the NL2HA-S714A point mutant (grey; n =12). P <0.05; Kolmogorov–Smirnov test. Note the shift to the right of the cumulative amplitude distribution curve obtained from cells transfected with the mutant as compared to controls. Full size image The selective increase in amplitude of sIPSCs detected in Pin1−/− mice suggest a post-synaptic site of action. This may involve an increase in the number of active GABA A Rs or changes in single-receptor channel conductance. To distinguish between these two possibilities, peak-scaled non-stationary fluctuations analysis of sIPSCs was performed only on stable recordings with no time-dependent changes in either peak amplitude, 10–90% rise time and decay time ( Fig. 8a ) (electrotonic filtering was excluded on the basis of no correlation between 10–90% rise time and decay time [30] ). Plotting the mean current amplitude versus variance and fitting individual points with the parabolic equation (equation (2) in the methods; Fig. 8b ), allowed estimating single-channel conductance and the number of channels open at the peak of spontaneous IPSCs. The single-channel conductance was calculated according to equation (3), assuming a reversal potential for chloride equal to 0. Interestingly, while the values of single-channel conductance were similar in both genotypes ( Fig. 8c ), the average number of active channels open at the peak of sIPSCs (Np) was significantly increased in Pin1−/− mice compared with controls (53±11 versus 26±5; P =0.03; Fig. 8c ). 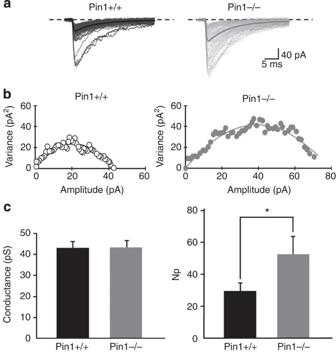Figure 8: Pin1 controls the number of active receptor channels at GABAergic synapses. (a) Individual sIPSCs from Pin1+/+ (black) and Pin1−/− mice (grey) are shown with the average currents (thick lines). (b) Current/variance relationships for sIPSCs shown ina(c) Summary plots of weighted mean channel conductance (43±3 pS and 43±3 pS,P=0.9, Student’st-test) and number of GABAAreceptor channels (Np) in wt (black;n=8) and in Pin1−/− mice (gray;n=5). *P=0.03, Student’st-test. Figure 8: Pin1 controls the number of active receptor channels at GABAergic synapses. ( a ) Individual sIPSCs from Pin1+/+ (black) and Pin1−/− mice (grey) are shown with the average currents (thick lines). ( b ) Current/variance relationships for sIPSCs shown in a ( c ) Summary plots of weighted mean channel conductance (43±3 pS and 43±3 pS, P =0.9, Student’s t -test) and number of GABA A receptor channels (Np) in wt (black; n =8) and in Pin1−/− mice (gray; n =5). * P =0.03, Student’s t -test. Full size image To further evaluate the possibility that higher amplitude inhibitory events recorded in Pin1−/− mice may originate from GABA A Rs containing different subunits, we measured in both genotypes the decay time constants of small and large amplitude events. Spontaneous IPSCs were plotted against their decay half-widths and arbitrarily divided in two main classes whose amplitude was <or>150 pA ( Fig. 9a , in green and blue, respectively). Notably, larger amplitude events (>150 pA) prevailed in Pin1−/− mice. No differences in decay of sIPSCs <or>150 pA were observed between Pin1+/+ and Pin1−/− mice, thus excluding the involvement of multiple receptor subtypes with different kinetics (the 90–10% decay ( τ ) of sIPSCs <150 pA was 9±1 ms in Pin−/− mice and 11±2 ms in Pin1+/+; P >0.05; τ of sIPSCs >150 pA was 11±2 ms in Pin−/− mice and 10±2 ms in Pin1+/+; P >0.05. The 90–10% decay time ( τ 90–10% ) of all sIPSCs was 11±2 ms and 10±2 ms in Pin1+/+ and Pin1−/− mice, respectively; Fig. 9b,c , P>0.05). These data altogether suggest that the observed increase in amplitude of sIPSCs in Pin1−/− mice is exclusively due a genuine increase in number of GABA A Rs composed of the same subunits. 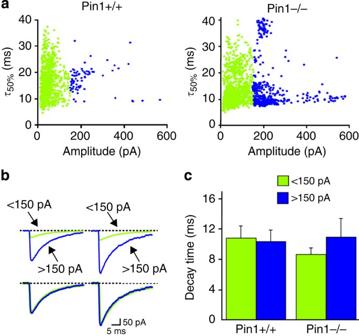Figure 9: Pin1 does not affect the decay kinetics of spontaneous IPSCs. (a) The peak amplitude of individual sIPSCs <150 pA (green) and >150 pA (blue) is plotted against their decay half-widths (τ50%) in Pin1+/+ and in Pin1−/− mice. (b) In the upper part, average traces of spontaneous IPSCs shown ina. In the lower part, average traces are normalized and superimposed. (c) Each column represents the mean 90–10% decay time constant of spontaneous IPSCs in Pin1+/+ and Pin1−/− mice, <150 pA (green),n=8 and 7, respectively and >150 pA (blue),n=6 and 7, respectively. For all comparisons,P>0.05, Student’st-test. Figure 9: Pin1 does not affect the decay kinetics of spontaneous IPSCs. ( a ) The peak amplitude of individual sIPSCs <150 pA (green) and >150 pA (blue) is plotted against their decay half-widths ( τ 50 %) in Pin1+/+ and in Pin1−/− mice. ( b ) In the upper part, average traces of spontaneous IPSCs shown in a . In the lower part, average traces are normalized and superimposed. ( c ) Each column represents the mean 90–10% decay time constant of spontaneous IPSCs in Pin1+/+ and Pin1−/− mice, <150 pA (green), n =8 and 7, respectively and >150 pA (blue), n =6 and 7, respectively. For all comparisons, P >0.05, Student’s t -test. Full size image GABA release and tonic inhibition are unaltered in Pin1−/− In a previous study, we demonstrated that the functional knockdown of NL2 was accompanied by a reduction in the probability of GABA release [31] , thus underlying the role of NLs as retrograde regulators of presynaptic function. Therefore, we evaluated here whether Pin1-dependent modulation of NL2–gephyrin interaction could also affect GABA release from presynaptic nerve terminals. To this end, we used 1,2,5,6-tetrahydropyridin-4-yl methylphosphinic acid (TPMPA), a low affinity competitive GABA A R antagonist [32] . This approach allowed to compare differences in presynaptic GABA transients between Pin1+/+ and Pin1−/− mice. Similar reduction of sIPSCs amplitude in both genotypes (51±6% versus 54±8%, P >0.05, Supplementary Fig. 3a,b ) was detected on bath application of TPMPA (200 μM), thus excluding a transsynaptic action of Pin1 on GABA release. Part of GABA released during synaptic activity may escape the cleft and invade the extracellular space to activate extrasynaptic high affinity GABA A Rs. This feature generates a persistent GABA A -mediated conductance [33] that is involved in a number of physiological processes [34] . To determine whether Pin1 signalling affects extrasynaptic GABA A Rs, we analysed the tonic GABA A -mediated conductance in both Pin1+/+ and Pin1−/−mice. The tonic conductance was assessed by the shift of the holding current induced by application of the GABA A R channel blocker PTX (100 μM) ( Supplementary Fig. 4a ). This drug caused a similar shift in holding current in Pin1−/− and Pin1+/+ mice ( Supplementary Fig. 4b,c ), indicating that extrasynaptic GABA A receptors are not influenced by Pin1-mediated signalling. The present study shows that NL2 is a newly identified substrate of proline-directed phosphorylation. This post-translational modification, acting on its unique Pin1 consensus motif localized within the CD (S714-P), modulates the amount of NL2–gephyrin complexes at synaptic sites. This modulation impacts on GABAergic transmission, by selectively affecting the total number of synaptic GABA A Rs. On the basis of these findings, post-phosphorylation prolyl-isomerization can play a crucial role in remodelling the GABAergic PSD to sustain plasticity processes. Protein phosphorylation on serine and threonine residues preceding a proline, the so-called proline-directed phosphorylation, has emerged as a mechanism regulating signalling events through conformational changes that are catalysed by the phospho-dependent recruitment of the peptidyl-prolyl isomerase Pin1. While the different roles of Pin1 in dividing cells have long been established and characterized [19] , its function in post-mitotic neurons in general and at synapses in particular is still poorly understood. In a previous study, we identified gephyrin, the main scaffolding protein of inhibitory PSD, as a new target of post-phosphorylation prolyl-isomerization [22] . Here, by inspecting the protein sequence of NL CDs, we identified S/T-P motifs that may provide Pin1 binding sites if phosphorylated in viv o. In particular, NL2 presents a unique Pin1 consensus site in its cytoplasmic region, S714-P, which is located 15 amino acids apart from the transmembrane domain. Even though this proximity to the plasma membrane raises doubts about its accessibility by a proline-directed kinase, several lines of evidence suggest that endogenous NL2 can undergo proline-directed phosphorylation. First, this isoform was recognized by the MPM2 antibody on NL2 immunoprecipitation from mouse brain homogenates. Second, MPM2-mediated NL2 immunoprecipitation was still maintained on removal of the NL2–gephyrin-binding domain, excluding the possibility of an indirect recognition mediated by endogenous gephyrin. Third, such detection was completely lost on NL2HA-S714A mutagenesis. This phosphorylation event is then able to directly recruit the effector molecule of the signalling cascade Pin1, as shown by co-immunoprecipitation experiments with endogenous neuronal proteins. Also in this case, Pin1 binding to NL2 was still maintained on the removal of the GBD, while it was completely abolished by mutating S714 to alanine, thus suggesting that the prolyl isomerase can be directly recruited by the unique NL2 Pin1 consensus motif in a phosphorylation-dependent manner. These results altogether indicate that NL2 represents a newly identified substrate for proline-directed signalling cascade in vivo. Our biochemical data demonstrate that NL2–gephyrin interaction is negatively regulated by proline-directed phosphorylation. Co-immunoprecipitation experiments on recombinantly expressed gephyrin-FLAG and NL2HA unveiled an enhanced complex formation on pharmacological inhibition of Pin1 catalytic activity. Similarly, endogenous NL2/gephyrin complexes pulled down from whole brain or hippocampal tissues of Pin1−/− animals were significantly augmented as compared with the corresponding WT tissues. These biochemical findings were also validated by immunocytochemistry performed on cultured hippocampal neurons, where we could detect a high number of clusters co-labelled for NL2 and gephryin as well as their increased apposition to presynaptic GABAergic inputs in the absence of Pin1 expression. Interestingly, the NL2 point mutant unable to undergo prolyl-isomerization was capable to recruit gephyrin even more efficiently as compared with the WT form, whereas gephyrin mutagenesis at two putative Pin1 consensus motifs, S270A and S319A, located within, or close to, the minimal NL2 binding domain, was completely ineffective. The fact that this post-translational modification seems to control the strength of NL2 association with gephyrin by acting mainly on NL2, and not vice versa , further reinforces the emerging idea that cell adhesion molecules are key determinant in regulating synapse function. In a recent study by Giannone et al . [18] , it has been demonstrated that the level of NL1 phosphorylation at a specific tyrosine residue located within the GBD dictates the strength of NL1/gephyrin interaction. In other words, NL1, the isoform enriched at excitatory synapses and therefore mostly associated with PSD95, can potentially recruit gephyrin as well as NL2, but its phosphorylation, promoted by neurexin–adhesion signalling, precludes such interaction while favouring PSD95 binding. Our experimental data indicate that proline-directed phosphorylation is acting similarly to tyrosine phosphorylation signalling. Since NL2 S714 is not positioned within the GBD, but is located just 50 amino acid upstream, it is reasonable to believe that Pin1-driven conformational changes, by affecting the overall folding of the CD, will induce gephyrin release ( Fig. 10 a). Alternatively, these conformational changes may promote NL2 tyrosine phosphorylation, an event shown to impede NLs/gephyrin interaction [18] ( Fig. 10 b). Interestingly, tyrosine to alanine mutagenesis on NL2 was shown to completely abolish recombinant gephyrin recruitment by the mutant protein or to strongly reduce its interaction with endogenous gephyrin [6] . Whether NL2 phosphorylation occurs at tyrosine 770 and whether this event is able to hamper gephyrin binding is still unknown. 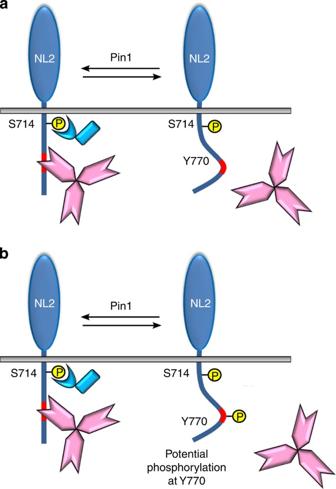Figure 10: Model of the putative cross-talk between proline-directed phosphorylation and tyrosine phosphorylation. Phosphorylation of NL2 CD at S714 by a proline-directed kinase allows the recruitment of the proly isomerase Pin1. Pin1-driven conformational changes, by altering the folding of the NL2 CD, may represent the main cause responsible for gephyrin detachment (a). Alternatively, Pin1-mediated structural rearrangement may render the conserved tyrosine residue of the GBD (Y770) susceptible to phosphorylation, an event shown to prevent NL1/gephyrin interaction (b). Figure 10: Model of the putative cross-talk between proline-directed phosphorylation and tyrosine phosphorylation. Phosphorylation of NL2 CD at S714 by a proline-directed kinase allows the recruitment of the proly isomerase Pin1. Pin1-driven conformational changes, by altering the folding of the NL2 CD, may represent the main cause responsible for gephyrin detachment ( a ). Alternatively, Pin1-mediated structural rearrangement may render the conserved tyrosine residue of the GBD (Y770) susceptible to phosphorylation, an event shown to prevent NL1/gephyrin interaction ( b ). Full size image The other partner of the complex is represented by gephyrin, a recognized target of Pin1 (ref. 22 ). Gephyrin contains 10 consensus motifs mostly concentrated in its C-domain, and all of them found to be phosphorylated in vivo [35] , [36] . This region of the protein is positioned between the amino-terminal G- and carboxyl-terminal E-domains, which are directly involved in gephyrin multimerization. Conformational changes induced by phosphorylation, possibly followed by prolyl-isomerization, are expected to alter the conformation of the gephyrin C-domain and in turn, regulate specific functional properties of gephyrin, in particular its binding to interacting proteins, including possibly NL2. However, the complexity of the system under investigation makes it very difficult to determine whether and how a specific phosphorylation event can contribute, directly or indirectly, to enhance gephyrin association to NL2. Nevertheless, it should be emphasized that gephyrin is robustly phosphorylated at several residues in vivo , thus suggesting that a specific pattern of phosphorylation, rather than a single post-translational modification, is functionally determinant. In contrast, NL2 possesses a unique target for prolyl-isomerization suggesting that it could represent the master switch of the signalling cascade. Our electrophysiological experiments clearly demonstrate that deletion of Pin1 specifically affects GABAergic transmission, causing a dramatic increase in amplitude, but not in frequency, of sIPSCs due to an increase in the number of GABA A Rs at post-synaptic sites. Notably, such enhancement was detected on neuronal overexpression of the NL2 mutant unable to undergo prolyl-isomerization, suggesting a functional link between the signalling cascade strengthening NL2/gephyrin interaction and the increased synaptic recruitment of GABA A Rs. There is a large body of evidence underlying the key role played by NL2 in promoting clustering and/or stabilization of GABA A Rs at post-synaptic sites. By employing a heterologous expression system, it was shown that GABA A Rs are able to co-aggregate with NL2 and only the presence of this isoform can induce strong GABAergic presynaptic differentiation from co-cultured neurons and promote the establishment of fully functional hemi-synapses [37] . In NL2-deficient mice, the number of functional GABA A Rs detected in the retina was shown to be drastically reduced [38] . Furthermore, targeting of GABA A Rs and gephyrin scaffold appeared severely compromised in the pyramidal cell layer of the CA1 region of the hippocampus, a morphological phenotype accompanied by a strong deficit in synaptic inhibition [6] . The increased recruitment of synaptic GABA A receptors in Pin1−/− mice may simply depend on the enhanced gephyrin targeting at synaptic sites. More scaffold deposition should offer a high number of binding sites available for the transient immobilization of GABA A Rs at inhibitory synapses. In addition, or alternatively, we cannot exclude the possibility that the extracellular domain of NL2 could also participate in GABA A Rs receptor recruitment. The unique S714-P consensus motif, located very close to the NL2 transmembrane domain, could influence the folding of the extracellular domain of NL2, rendering it incapable to interact in cis with GABA A R subunits. This type of mechanism has been shown to operate at excitatory synapses, where the abundance of NMDARs is controlled by the interaction occurring between the GluN1 subunit with NL1-specific sequences located in its extracellular domain [39] . In conclusion, our findings unveil the existence of a new signalling pathway operating at GABAergic synapses to alter the efficacy of GABAergic transmission by modulating NL2/gephyrin interaction. Although a comprehensive understanding of the molecular mechanisms underlying the action of Pin1 on NL2/gephyrin interaction is still lacking, we believe that our study further emphasizes the key role played by NL2 in organizing and stabilizing GABAergic synapses. Plasmid constructs The expression construct for HA-tagged human NL2 in pNice was kindly provided by P. Scheiffele (Biozentrum, Basel). The amino acid sequence ranging from residues 768 to 782 was removed to generate the NL2HA lacking the gephyrin binding domain (pNice-NL2HA-ΔGBD). S714A mutation was also introduced into pNice-NL2HA-ΔGBD to remove the unique Pin1 consensus site (pNice-NL2HA-ΔGBDS714A). All PCR-based mutagenesis were fully sequenced to exclude the possibility of second site mutations. pcDNA3-FLAG-Pin1 WT and pcDNA3-gephyrin-FLAG have been previously described [22] . EGFP-tagged gephyrin point mutants (S270A and S319A), the WT and the truncated version ranging from amino acid 326 to 736 and 310 to 736, were PCR cloned into the Xho I/ Hin dIII sites of pEFP-C1 (Clontech, Mountain View, CA). EGFP-tagged gephyrin GC (1–310) was kindly provided by G. Schwarz (University of Cologne, Germany) [40] . Cell cultures and transfections HEK-293-T cells were cultured at 37 °C under a 5% CO2 atmosphere in Dulbecco’s modified Eagle’s medium supplemented with 10% fetal bovine serum. They were transiently transfected with various plasmid constructs using Lipofectamine 2000 (Invitrogen) according to the manufacturer’s protocol. Cells were collected 24–48 h after transfection. Primary hippocampal neurons from P0 Pin1+/+ and Pin1−/− littermates and rat hippocampal neurons were prepared as previously described [41] . Being Pin1−/− mice infertile, Pin1+/+ and Pin1−/− littermates for neuronal cultures were routinely obtained by mating heterozygous mice [42] . Each hippocampus derived from single newborn littermate was processed and plated separately and identified by tail genotyping. Neurons were Lipofectamine transfected after 8 DIV with 1 μg of EGFP-gephyrinWT or EGFP-gephyrinS270A and processed for immunofluorescence 2–3 days later. For electrophysiological recordings, neurons were co-transfected with 1 μg NL2HA/NL2HA-S714A and 500 ng of green fluorescent protein (GFP) to visualize transfected cells. PiB treatments To inhibit Pin1 catalytic activity, the chemical inhibitor PiB (diethyl-1,3,6,8-tetrahydro-1,3,6,8-tetraoxobenzol-phenanthroline-2,7-diacetate) was added to the culture medium for 24 h at a concentration of 2.5 μm. PiB was purchased from Calbiochem and resuspended in DMSO. Immunoprecipitation and chemical cross-linking Immunoprecipitation for MPM2 experiments was performed using a lysis buffer containing 50 mM Tris–HCl, pH 7.5, 1% Nonidet P-40, 0.5% Triton X-100, 150 mM NaCl, 1 mM Na 3 VO 4 , 50 mM NaF and protease inhibitor mixture (Sigma). For NL2HA and gephyrin co-immunoprecipitation, HEK293 cells overexpressing NL2HA and gephyrin-FLAG were treated 48 h after transfection with 2.5 mM PiB or mock treated with DMSO as negative controls. Cells were lysed in 50 mM Tris-HCl, pH 7.5, 100 mM NaCl, 0.1% Tween 20, 10% glycerol, 10 mM EDTA, 2 mM MgCl 2 and protease inhibitor mixture and immunoprecipitated by either the anti-FLAG antibody or anti-HA agarose (Pierce). Co-immunoprecipitation of native gephyrin–NL2 complexes from p15 Pin1+/+ and Pin1−/− mouse brains or hippocampal tissues was performed using a chemical cross-linking approach on postnuclear homogenates as previously described [6] . Primary antibodies were revealed by HRP-conjugated secondary antibodies (Sigma) followed by ECL (Amersham Biosciences). Biotinylation assay and analysis on synaptosomes To examine changes in NL2 transported at the plasma membrane, we performed biotinylation assays on hippocampal neuronal cultures derived from Pin1+/+ and Pin1−/− mice. Neuronal cells were incubated with 0.5 mg ml −1 EZ-Link Sulfo-NHS-LC-Biotin (Pierce) in PBS at 4 °C for 30 min. To quench the reaction, cells were washed three times with cold PBS containing 0.1 M Tris-HCl pH 7.4. Cells were then lysed in lysis buffer containing protease inhibitor cocktail followed by centrifugation at 1,000 g for 5 min. The collected lysate were incubated with streptavidin cross-linked to agarose beads (Pierce) for 2 h at 4 °C. The beads were then washed twice with lysis buffer, and eluted with SDS loading buffer. The amount of membrane protein loaded in each experiments was normalized to the amount of the glycophosphatidylinositol-anchored protein Flotilin1, whose expression levels are identical in both mouse genotypes. PSD enriched extracts were prepared by using the Syn-PER Synaptic Protein Extraction Reagent (ThermoScientific) following the manufacturer’s instructions. Briefly, a pool of four hippocampi derived from the same genotypes were homogenized in the Extraction reagents (10 ml of reagent per g of tissue), centrifuged at 1,200 g for 10 min. The pellet was discarded while the supernatant (homogenate) was additionally centrifuged at 15,000 g for 20 min. The cytosolic fraction was discarded and the pellet containing the synaptosomes was resuspended in 400–500 μl of reagent and analysed by western blot analysis. The protein concentration of each sample was determined using the Pierce BCA Protein Assay to allow an equal loading of total protein. Western blot analysis Western blot image acquisition was performed using the ECL detection kit and the Alliance 4.7 software (UVITECH, Cambridge). Quantifications were performed using the UVIband imager software (Amersham). The relative amount (Input, 1/20 of the total lysate) of the different antigens considered in this study and the immunoprecipitated fractions were determined by densitometry on the acquired images. The amount of immunoprecipitated and coimmunoprecipitated proteins are first normalized to their corresponding inputs and then the coimmunoprecipated value is additionally normalized on the immunoprecipitated antigen. Full images of western blots are in Supplementary Fig. 5 . Antibodies The following antibodies were used in immunohistochemistry and immunocitochemistry: anti-gephyrin Mab7a (Synaptic System Cat. No 147021), anti-VGAT rabbit or guinea pig (1:1,000, Synaptic System Cat. No 131004), anti-NL2 rabbit affinity purified (1:500, Synaptic system Cat, No 129203), guinea pig anti-GABA A γ2 subunit (1:2,000 (ref. 43 )), biotinylated anti-guinea pig (1:200, Vector Laboratories, Cat No BA-7000). The following primary antibodies were used in immunoprecipitation and western blot analysis: mouse monoclonal anti-FLAG M2 (Sigma Cat No F1804), mouse monoclonal anti-gephyrin 3B11 (Synaptic System Cat No 147111) and rabbit polyclonal anti-NL2 (Synaptic Systems Cat. No 129202), pS/pT-P (MPM2, Upstate Biotechnology Cat No 05-368), high affinity rat monoclonal anti-HA 3F10 (Roche), anti-GFP rabbit monoclonal (Life Technology, Cat No G10362). Validation of antibodies used in these assays can be found on the respective manufacturers' websites. Immunohistochemistry and immunocytochemistry Eight-week-old Pin1+/+ and Pin1−/− littermates (for each genotype, n =3) were anaesthetized and perfused transcardially with 0.1 M phosphate buffer, pH 7.4 (PB). Brains were quickly removed from the skull and frozen with isopentane cooled to −40 °C with liquid nitrogen. Ten to 12-μm thick cryostat sections were collected on Superfrost glass slides and further processed for immunostaining for combined detection of VGAT and GABAA γ2 or VGAT and gephyrin. Briefly, cryostat sections were fixed by immersion in 2% paraformaldehyde, and mildly treated with pepsin as antigen-retrieval procedure, and then incubated for 48 h with different combination of primary antibodies. Secondary antibody staining was performed for 1 h at room temperature using anti-isotypic fluorophore-conjugated antibodies Alexa-488 and Alexa-594 at dilutions of 1:1,000 (Molecular Probes). Hippocampal neurons grown on glass coverslips were fixed with 4% paraformaldehyde and 4% sucrose in PBS. Unspecific binding was blocked by incubation with 10% normal goat serum in PBS. Primary and secondary antibodies were diluted in 5% normal goat serum/PBS. Secondary antibodies included anti-isotypic fluorophore conjugated antibodies Alexa-488, Alexa-594 and streptavidin-Alexa 405 at dilutions of 1:1,000 (Molecular Probes). Confocal microscopy and image analysis Fluorescence images were acquired on a TCS-SP confocal laser scanning microscope (Leica, Bensheim, Germany) with a × 40 1.4 NA or × 63 1.4 NA oil immersion objectives, additionally magnified fivefold with the pinhole set at 1 Airy unit. All the parameters used in confocal microscopy were consistent in each experiment, including the laser excitation power, detector and off-set gains and the pinhole diameter. Stacks of z-sections (12–13 optical sections) with an interval of 0.3 μm were sequentially scanned three times for each emission line to improve the signal/noise ratio. The number of gephyrin, γ2 subunit and VGAT puncta was assessed in at least eight sections for each genotypes (Pin1+/+ and Pin1−/−), by taking at least four images of strata radiatum and oriens of the CA1 region of each hippocampus in each set of experiments ( n =3). In the pyramidal cell layer, the high density and elongated shape of VGAT positive terminals precluded the determination of their numbers and their colocalization with the other two antigens investigated. For immunocitochemistry samples, at least 10 cells from at least three independent batches per condition were used for analysis. Images were acquired as a z -stack (six to seven optical sections, 0.25 μm step size). In each image, at least five dendritic segments were outlined and saved as regions of interest. Quantification of immunofluorescence data was performed using the Volocity3D Image Analysis Software (PerkinElmer, London, UK). Gephyrin, NL2, GABA A R γ2 and VGAT clusters were determined after thresholding of images. Thresholds were determined using the ‘voxel spy’ facility of the software and chosen such that all recognizable punctuate structures were included into the analysis (minimal area, 0.1 μm 2 ); colocalization was evaluated based on the determination of thresholded Pearson’s correlation coefficient (PCC>0,5) for each gephyrin and γ2 cluster previously identified and quantified [44] . NL2 colocalization with gephyrin puncta was also quantified utilizing the software function ‘intersect object’ that measures size, volume and intensity values of intersecting objects identified by separate protocols in each channel. To determine the degree of apposition of NL2/gephyrin colabeled clusters with the presynaptic marker VGAT, we superimposed the mask of all identified overlapping puncta onto the third channel and count them manually. Hippocampal slice preparation and drug treatment All experiments were performed in accordance with the European Community Council Directive of November 24, 1986 (86/609EEC) and were approved by the local authority veterinary service and by SISSA ethical committee. All efforts were made to minimize animal suffering and to reduce the number of animal used. Transverse hippocampal slices (300 μm thick) were obtained from postnatal (P) day P10–P13 mice (male and female) using a standard protocol [45] . Briefly, after being anaesthetized with CO 2 , animals were decapitated. The brain was quickly removed from the skull and placed in ice-cold artificial cerebrospinal fluid containing (in mM): 130 NaCl, 25 glucose, 3.5 KCl, 1.2 NaH 2 PO 4 , 25 NaHCO 3 , 2 CaCl 2 and 1.3 MgCl 2 , saturated with 95% O 2 and 5% CO 2 (pH 7.3–7.4). Transverse hippocampal slices (300 μm thick) were cut with a vibratome and stored at room temperature (22–24 °C) in a holding bath containing the same solution as above. After incubation for at least 45 min, an individual slice was transferred to a submerged recording chamber and continuously superfused at 33–34 °C with oxygenated artificial cerebrospinal fluid at a rate of 3–4 ml min −1 . The following drugs were used: DNQX, PTX and bicuculline, purchased from Ascent Scientific; TPMPA purchased from Tocris Bioscence. DNQX and PTX were dissolved in DMSO. The final concentration of DMSO in the bathing solution was 0.1%. At this concentration, DMSO alone did not modify the membrane potential, input resistance or the firing properties of CA1 pyramidal neurons. Drugs were applied in the bath by gravity via a three-way tap system by changing the superfusion solution to one differing only in its content of drug(s). The ratio of flow rate to bath volume ensured a complete exchange within 2 min. Electrophysiological recordings Whole-cell patch-clamp recordings (in voltage clamp configuration) were performed from CA1 pyramidal cells, visualized with an upright microscope equipped with differential interference contrast optics and infrared video camera, using a patch-clamp amplifier (Axopatch 1D amplifier, Molecular Devices, Sunnyvale, CA, USA). Patched electrodes were pulled from borosilicate glass capillaries (Hingelberg, Malsfeld, Germany). They had a resistance of 4–6 MΩ when filled with the intracellular solution containing (in mM): 125 Cs-methanesulphonate, 10 CsCl, 10 HEPES, 0.3 EGTA, 2 MgATP, 0.3 NaGTP (pH adjusted to ~7.3 with CsOH; the osmolarity was adjusted to 290 mOsmol). The stability of the patch was checked by repetitively monitoring the input and series resistance during the experiment. Cells exhibiting >20% changes in series resistance were excluded from the analysis. The series resistance was <25 MΩ and was not compensated. Spontaneous GABAergic (sIPSCs) and glutamatergic (sEPSCs) post-synaptic currents were routinely recorded from a holding potential of −60 mV in the presence of DNQX (20 μM) and PTX (10 μM), respectively. While sEPSCs were recorded using patch pipettes filled with the above mentioned solution, sIPSCs were recorded using an intracellular solution containing (in mM): CsCl 137, Hepes 10, BAPTA 11, MgATP 2, MgCl 2 2, CaCl 2 1 and 5 QX-314 (pH adjusted to ~7.3 with CsOH). sIPSC were also recorded from cultured hippocampal neurons co-transfected with GFP and NL2HA or NL2HA-S714A 24 h after transfection, at a holding potential of −60 mV in presence of DNQX (20 μM) with the same intracellular solution used for the acute slices experiment. The extracellular solution contained (in mM) 137 NaCl, 5 KCl, 2 CaCl 2 , 1 MgCl 2 , 20 glucose and 10 HEPES, pH 7.4 (corrected with NaOH). Data analysis Data were acquired and digitized with an A/D converter (Digidata 1,200, Molecular Devices) and stored on a computer hard disk. Acquisition and analysis were performed with Clampfit 9 (Molecular Devices). Data were acquired at 20 kHz, filtered with a cut-off frequency of 2 kHz and stored on computer hard disk to perform off-line analysis. The resting membrane potential was measured immediately after break-in and establishing whole-cell recording. The membrane input resistance ( R in ) was calculated by measuring the amplitude of voltage responses to steady hyperpolarizing current steps, using the Clampfit 10.0 program (Molecular Devices). Spontaneous AMPA- and GABA A -mediated post-synaptic currents were analysed using Clampfit 10.0 (Molecular Devices). This programme uses a detection algorithm based on a sliding template. The template did not induce any bias in the sampling of events because it was moved along the data trace by one point at a time and was optimally scaled to fit the data at each position. The detection criterion was calculated from the template-scaling factor and from how closely the scaled template fitted the data. Spontaneous GABAergic currents were analysed with Mini Analysis program (version 6.0.1, Synaptosoft, Leonia, NJ) for their decay time constants. Only events with no deflections in the rising or decaying phases were included in the analysis. Low amplitude (<5 pA) events as well as events whose amplitude correlated with the rising or decaying time constants were discarded from the analysis because they were thought to be affected by dendritic filtering. The decay time of s IPSCs were fitted with a single exponential function as: where I(t) is the current as a function of time, A is the amplitude at time 0, τ is the time constant. The Mini Analysis programme was used to perform peak-scaled non-stationary noise analysis according to Traynelis and co-workers [46] . Individual, not correlated, events were aligned to the point of steepest rise time. The peak of the mean current response waveform was scaled to the response value at the corresponding point in time of each individual event before subtraction to generate the difference waveforms. The ensemble mean post-synaptic current was binned into 50 bins of equal amplitude to assign similar weights to all phases of ensemble mean waveform. Variance was plotted against amplitude and individual points were fitted with the equation: where i is the unitary single-channel current, I is the mean current, N is the number of channels open at the current peak and σ b 2 is the variance of the background noise. The single-channel chord conductance ( ) was calculated as: from the holding potential ( E m ) of −60 mV, assuming a reversal potential ( E rev ) of 0 mV. Amplitude distribution of sIPSCs amplitude was obtained fitting data with the following Gaussian function: where I σ is the mean current, a i is the area and σ is the variance. The amplitude of the tonic current was estimated by the outward shift of the baseline current after the application of the GABA A receptor channel blocker PTX (100 μM). Only current recordings that exhibited a stable baseline were included in the analysis. Baseline currents were estimated by plotting four to five 0.5 s periods in all point histograms. These were fitted with a Gaussian function. The peak of the fitted Gaussian was considered as the mean holding current [47] . Statistics Statistical analyses for Co-IP, PSD enriched extracts fractions analyses were performed by using Microsoft Excel. Comparisons were performed by Student’s t -test two-tailed distribution unequal variance. Deviation and error bars were calculated using the same software. Statistical significance was defined as P <0.05. Statistical analyses of morphological data (NL2 and gephyrin cluster size and density) were performed pair-wise (Pin1−/− versus Pin1+/+) using unpaired, two-tailed Student’s t -test. Bars indicate (s.d.) Statistical analyses for electrophysiological experiments were performed by using pClamp 10 and Microsoft Excel. Comparison were perfomed by Student’s t -test unless otherwise stated. Statistical significance was defined as P <0.05. How to cite this article: Antonelli, R. et al . Pin1-dependent signalling negatively affects GABAergic transmission by modulating neuroligin2/gephyrin interaction. Nat. Commun. 5:5066 doi: 10.1038/ncomms6066 (2014).